Sema3E/PlexinD1 regulates the migration of hem-derived Cajal-Retzius cells in developing cerebral cortex During the development of the cerebral cortex, Cajal-Retzius (CR) cells settle in the preplate and coordinate the precise growth of the neocortex. Indeed, CR cells migrate tangentially from specific proliferative regions of the telencephalon (for example, the cortical hem (CH)) to populate the entire cortical surface. This is a very finely tuned process regulated by an emerging number of factors that has been sequentially revealed in recent years. However, the putative participation of one of the major families of axon guidance molecules in this process, the Semaphorins, was not explored. Here we show that Semaphorin-3E (Sema3E) is a natural negative regulator of the migration of PlexinD1-positive CR cells originating in the CH. Our results also indicate that Sema3E/PlexinD1 signalling controls the motogenic potential of CR cells in vitro and in vivo . Indeed, absence of Sema3E/PlexinD1 signalling increased the migratory properties of CR cells. This modulation implies negative effects on CXCL12/CXCR4 signalling and increased ADF/Cofilin activity. Cajal-Retzius cells (CR) are early generated neurons located in the preplate during early cortical development and, later in development, in the perinatal marginal zone-layer I (see refs 1 , 2 for reviews). These pioneer cells have been largely studied in rodents, feline, primates and human (see refs 3 , 4 , 5 , 6 , 7 ). These studies reported that, in mouse neocortex, CR cells largely disappeared during the first postnatal week by programmed cell death [6] , [8] . During corticogenesis, CR cells seem to play several roles: modulating appropriate migration of cortical plate neurons, actively participating in neuronal network activity in developing marginal zone/layer I, with the capacity to generate action potentials, establishing synaptic contacts in the marginal zone/layer I and receiving excitatory and GABAergic inputs [9] , [10] , [11] . Mouse CR cells are mainly generated in the cortical hem (CH), the septum/retrobulbar area, and the pallial/subpallial boundary [2] , [12] . Shortly after generation, CR cells migrate through the preplate/marginal zone to populate the entire cortical surface following a specific rostrocaudal and lateral tangential process [12] , [13] , [14] . Birthdates of cortical CR cells are between embryonic days 8.5–13.5 (E8.5–13.5) in the mouse with a maximum between E9.5 and E12.5 (refs 6 , 15 ). For CR cells localized in the hippocampal region, this generation peaks around E11.5 (ref. 16) [16] . Genetic screening of CR cells has revealed that a large number of factors are involved in their generation, migration and maturation, such as p73 , p21 , Zic1-3, Lhx5 and Fgf8 , Tbr1 and 2 , Pax6 , Emx1 and Emx2 , Dbx1 , Foxg1 , Ebf2, Foxc1, LIM-homeobox genes, and miRNA9 among others (see references in refs 1 , 2 ). Concerning migration, there are not many molecules identify as regulators of CR cells migration. The chemokine CXCL12 (also known as SDF1) expressed by meningeal cells has been found to be mainly responsible for hem-derived CR cell migration [17] , [18] as occurs with other neural populations [19] . However, a study by Zarbalis et al. [20] , analysing hypomorphic Foxc1 mice with meningeal deficits suggests that meningeal as well as additional non-meningeal factors may modulate the migration of Reelin-positive cortical CR cells in the preplate. Indeed, a recent study reveals that their distribution in the marginal zone/layer I is modulated by contact-repulsive actions mediated by Eph/ephrin mechanisms [14] . In addition, there are evidences that confirm that CR cells expressed nectin1 that mediates heterotypic interactions with nectin3 in the leading processes of migrating projection neurons. The interactions between both nectins control radial migration by acting in concert with Reelin and Cdh2 to promote interactions between migrating neurons and CR cells [21] . The activity of CXCL12 and its receptors has been found to play a role in controlling the migration of other cortical neurons (for example, GABAergic interneurons) that are also influenced by the action of Semaphorins and their receptors [22] , [23] . Semaphorins and their receptors, Plexins and Neuropilins, have emerged as important cellular cues regulating key developmental processes, as neuronal migration and axonal guidance [24] . However, their participation in the migration of CR cells remains unknown. Regarding this challenging question, it is interesting that there are several articles that connect CXCL12 with semaphorins in neural and immune cell migration [25] . Today, it is generally accepted that blood vessels and nerves are structurally similar complex branched systems in the developing and adult brain [26] . Angiogenic factors, especially vascular endothelial growth factor (VEGF), are now known to play roles in neurogenesis and migration [27] . Endothelial tip cells guide outgrowing capillaries in response to gradients of extracellular, matrix-bound VEGF. In addition to VEGF, several axon guidance molecules, including Semaphorins, Netrins, Ephrins and Slits, have also been implicated in blood vessel pathfinding and capillary network formation [26] , [28] . In particular, Semaphorin-3E (Sema3E) and its receptor PlexinD1 have recently been shown to direct endothelial tip cell navigation, reinforcing the notion of shared mechanisms between neuronal and blood vessel pathfinding [28] , [29] . In the present study, we demonstrated that Sema3E/PlexinD1 signalling also participates in the regulation of CR cell migration. Indeed, PlexinD1 is expressed by CH-derived murine CR cells throughout their lives. More importantly, signalling mediated by Sema3E/PlexinD1 might modulate the migration of CR cells by decreasing CXCL12/CXCR4 signalling and increasing ADF/Cofilin activation, leading to control of their motogenic properties. Indeed, the absence of Sema3E/PlexinD1 signalling leads to changed CR cell distribution in marginal zone/layer I throughout the developing neocortex. Murine CR cells express PlexinD1 Using a microdissection procedure and further gene expression analysis performed on developing hippocampi, we determined that Plxnd1 expression is enriched in the stratum lacunosum-moleculare (slm) compared with other hippocampal layers of the cornus ammonis 1 (CA1) at perinatal stages in C57BL/6J mice (1.5±0.02 fold increase in reverse transcriptase quantitative PCR (RT–qPCR) values, control values of slm genes: Reln, 2.1±0.02 or Gdf5 1.23±0.02 in contrast to Sema3E (−1.15±0.02 fold decrease; mean±s.e.m.) ( Supplementary Fig. 1 ). Parallel in situ hybridization analysis determined that the Plxnd1 expression in the hippocampal slm/ml closely matched (Reelin) Reln messenger RNA (mRNA) and Calretinin (CALR)-positive cells distribution at P0 ( Supplementary Fig. 1 ). Plxnd1 distribution was also complementary to Sema3E expression present in the principal neurons of CA1-3 of the hippocampus proper and in granule cells of the dentate gyrus ( Supplementary Fig. 1 ; see also ref. 30 ). Next, we aimed to determine whether PlexinD1 is also expressed in CH-derived CR cells of the cortex in the earliest stages (E12.5) of corticogenesis (at the end of the preplate stage) as well as in the perinatal stages (P0) ( Fig. 1 and Supplementary Fig. 2 ). To ascertain this, we conducted three sets of experiments. First, we performed non-radioactive in situ hybridization experiments with Plxnd1 -specific probes ( Fig. 1a,d ); second, we performed single immunoperoxidase ( Supplementary Fig. 2 ) and double fluorescence immunostaining of CR cells at postnatal day 0 (P0) using antibodies against Reelin, CALR and eGFP, as reporter in Plxnd1 -eGFP mice ( Fig. 1g–o ). Finally, binding experiments were done of unfixed freshly prepared E12.5 telencephalic brain sections, using Sema3E-AP ( Supplementary Fig. 2d ). Results indicated that the pattern of Plxnd1 and Sema3E expression in developing pallial and subpallial regions at E12.5 was as recently reported [31] ( Fig. 1 ). However, in developing mouse neocortex, these approaches also showed that PlexinD1 was present in blood vessels but more relevantly in CR cells in the marginal zone/layer I ( Fig. 1 , see also Supplementary Fig. 2 ). In contrast, Plxnd1 mRNA signals, eGFP staining and tissue-binding Sema3E-AP labelling were absent in the CH. Moreover, detailed analysis of Plxnd1 -eGFP showed that all eGFP-positive cells and processes in the marginal zone were double labelled with Reelin or CALR, which ruled out the expression of Plxnd1 in neurons other than CR cells in this layer at these developmental stages in dorsal pallium ( Fig. 1g–o ). In addition, Sema3E mRNA detection was absent in the upper cortical layers as well as in meningeal cells and blood vessels ( Fig. 1b,e ). However, the presence of the Sema3E protein was detected in the upper neocortical layer using western blotting techniques ( Supplementary Fig. 3 ). Moreover, revealed sections suggested that Sema3E mRNA is more expressed in dorsomedial than in lateral neocortical regions (arrows in Fig.1b ), as well as being of note in the ventricular region of the subpallium (lateral ganglionic eminence and medial ganglionic eminence) (arrowheads in Fig. 1b ). 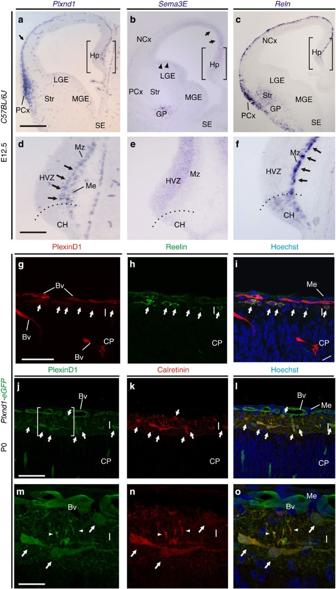Figure 1: mRNA distribution ofPlxnd1and Sema3Ein the developing telencephalon. (a–f) Distribution ofPlxnd1, Sema3EandRelnmRNAs in the mouse telencephalon at E12.5.Plxnd1expression was observed in the piriform cortex (PCx) and the lateral regions of the cortical plate (CP, arrow ina) as well as in the meninges (Me) and CR cells (arrows ind).Sema3Ewas observed in the globus pallidus (GP) (b) as well as in the ventricular/subventricular zone of the dorsal neocortex (NCx) and hippocampus (Hp) (b,e). Relnwas observed in the striatum (Str), PCx and throughout the cortical marginal zone (MZ) (arrows inf). The boxed area in (a–c) is shown in (d–f) at higher magnification. Note that some CH cells (dashed line) expressedRelnin these embryonic stages. (g–o) PlexinD1 was expressed by cortical CR cells. Double fluorescence images for Reelin and PlexinD1 in the upper neocortical layers (g–i). (j–o) Pictures showed double labelling of the upper neocortical layers ofPlxnd1-eGFP mice at P0 (eGFP,j,l,m,oand Calretinin (CALR),k,n,l,o). Meningeal blood vessels (Bv) as well as CR cells in layer I (arrows ing,I,j,l,m,o) were labelled with eGFP/PlexinD1 antibodies. Only CR cells were stained using Reelin or CALR immunostaining (h,i,k,l,n,o). The boxed region injis shown at higher magnification inj–l. Note the characteristic thin dendritic appendages (arrowheads inm–o) ascending towards the pia. HVZ, hippocampal ventricular/subventricular region; LGE–MGE, lateral and medial ganglionic eminences; SE, Septal region. Scale bars, 300 μm ina–c; 150 μm ind–f; 75 μm ing–l; 50 μm inm–o. Figure 1: mRNA distribution of Plxnd1 and S ema3E in the developing telencephalon. ( a – f ) Distribution of Plxnd1 , S ema3E and Reln mRNAs in the mouse telencephalon at E12.5. Plxnd1 expression was observed in the piriform cortex (PCx) and the lateral regions of the cortical plate (CP, arrow in a ) as well as in the meninges (Me) and CR cells (arrows in d ). Sema3E was observed in the globus pallidus (GP) ( b ) as well as in the ventricular/subventricular zone of the dorsal neocortex (NCx) and hippocampus (Hp) ( b , e ) . Reln was observed in the striatum (Str), PCx and throughout the cortical marginal zone (MZ) (arrows in f ). The boxed area in ( a – c ) is shown in ( d – f ) at higher magnification. Note that some CH cells (dashed line) expressed Reln in these embryonic stages. ( g – o ) PlexinD1 was expressed by cortical CR cells. Double fluorescence images for Reelin and PlexinD1 in the upper neocortical layers ( g – i ). ( j – o ) Pictures showed double labelling of the upper neocortical layers of Plxnd1 -eGFP mice at P0 (eGFP, j , l , m , o and Calretinin (CALR), k , n , l , o ). Meningeal blood vessels (Bv) as well as CR cells in layer I (arrows in g , I , j , l , m , o ) were labelled with eGFP/PlexinD1 antibodies. Only CR cells were stained using Reelin or CALR immunostaining ( h , i , k , l , n , o ). The boxed region in j is shown at higher magnification in j – l . Note the characteristic thin dendritic appendages (arrowheads in m – o ) ascending towards the pia. HVZ, hippocampal ventricular/subventricular region; LGE–MGE, lateral and medial ganglionic eminences; SE, Septal region. Scale bars, 300 μm in a – c ; 150 μm in d – f ; 75 μm in g – l ; 50 μm in m – o . Full size image At later embryonic stages (E14.5–E16.5) neuronal PlexinD1 labelling follows a lateral to medial gradient of expression that is relevant in neurons of the emerging cortical plate (from E12.5–E14.5) and in subplate cells of lateral regions of neocortex but not medial portions, especially at E16.5 ( Supplementary Fig. 2 ). This observation largely supports recent data indicating that subplate cells express Plxnd1 shortly after being split from the preplate to the subplate [31] . At developing subpallium, labelling of PlexinD1 remained as in previous stages with a relevant increase in staining in the striatum and in the anterior commissure ( Supplementary Fig. 2c ). More importantly, after birth, the number of CR cells (eGFP positive) in layer I decreased considerably during the first postnatal week, in line with the natural fate of this cellular population in mice [6] ( Supplementary Fig. 4 ). Indeed, aberrant shapes of double-labelled cells (eGFP-CALR) were observed at P0 but especially at P5 ( Supplementary Fig. 4b,d ). These morphologies with shrunken dendrites and fragmented perikarya have been associated with dying CR cells at these stages [6] . Sema3E influences CR cell migration via PlexinD1 Next we aimed to explore whether Sema3E/PlexinD1 modulates CH-derived CR cell migration ( Fig. 2 ). To determine this, we cultured CH from E12.5 Plxnd1 -eGFP embryos in three-dimensional hydrogels that were further treated with Sema3E-AP or secreted alkaline phosphatase (SEAP)-conditioned media ( Fig. 2a–f ), or which were, alternatively, confronted for 24–36 h in culture with COS1 cell aggregates secreting Sema3E-AP or SEAP ( Supplementary Fig. 5a,b,e ). Analysis of immunoreacted explants demonstrated eGFP ( Fig. 2b ) or PlexinD1 expression ( Fig. 2c ) in migrating CR cells. Numerous cells migrated radially from the CH explants in SEAP-treated cultures ( Fig. 2d,f and Supplementary Fig. 4a,e ). However, cultures treated with Sema3E-AP-conditioned media, as well as those confronted with Sema3E-AP-secreting COS1 cell aggregates, displayed low numbers of migrating cells compared with controls ( Fig. 2e,f and Supplementary Fig. 5b,e ). More importantly, no differences in the trajectory of migrating neurons were observed in confrontation experiments between groups (for example, CH versus COS1 secreting Sema3E-AP; ratio QP/QD SEAP: 1.08±0.11; Sema3E-AP: 0.91±0.12; mean±s.e.m. ), suggesting a motogenic rather than a chemotropic effect of Sema3E-AP in hem-derived CR cells ( Fig. 2d,e ; see also Supplementary Fig. 5 ). These results were corroborated by video time-lapse analysis of migrating CR cells in explant cultures. In these experiments, a significant decrease of 32.5% of migrated distance of identified CR cells from the CH was observed in the presence of Sema3E-AP compared with SEAP-treated explants ( Fig. 2g–k , Supplementary movies 1–4 ). Although we observed this change in migrating CR cells in our video time-lapse experiments, differences in the number of migrating cells were not associated with either decreased proliferation or increased cell death in CH explants ( Supplementary Fig. 5 ). Next, to determine whether the AP flag may affect to CR cells migration, we repeated the experiments by adding Sema3E-myc to the culture medium with similar results. In addition, we also want to answer if other members of class 3-secreted Semaphorins could also trigger similar effects in vitro , particularly Sema3A and Sema3F, which have been implicated in the migration of other cortical neurons (for example, GABAergic interneurons; see above) ( Supplementary Fig. 5 ). Results demonstrated that Sema3E-AP or -myc reduced the number and the migrated distance of CH-derived CR cells in our experiments ( Supplementary Fig. 5 ). 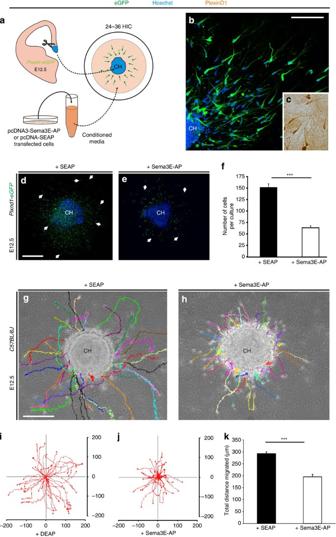Figure 2: Sema3E decreases hem-derived CR cell migrationin vitro. (a) Schematic representation of the experimental design. (b,c) Example of CR cells migrating from E12.5 hem explants ofPlxnd1-eGFP mice immunoreactive for eGFP (b) and PlexinD1 (c). (d–f) Comparison of CR cells migration (arrows ind,e) after incubation with SEAP (d) and Sema3E-AP (e) in E12.5 CH explants ofPlxnd1-eGFP. Quantifications of the experiments are shown inf. Plots show mean±s.e.m. SEAP (n=14); Sema3-AP (n=18). ***P<0.001, Student’st-test. (g,h) Examples of identified CH-derived CR cells migration on SEAP (g) and Sema3E-AP (h) treated cultures. Each CR cell trajectory is labelled with a different colour line using the (ImageJ) software analysis. (I,j) Graph showing the trajectories of identified CR cells in the video time-lapse experiments. A total of 38 and 39 cells are plotted iniandj, respectively. (k) Histogram showing the total distance migrated in the video time-lapse experiments and the effect of the Sema3E-AP incubation. Data are represented by mean±s.e.m. of three different experiments. ***P<0.001 Student’st-test. Scale bars,b=200 μm pertains toc.d=300 μm pertains toe,gandh. Figure 2: Sema3E decreases hem-derived CR cell migration in vitro . ( a ) Schematic representation of the experimental design. ( b , c ) Example of CR cells migrating from E12.5 hem explants of Plxnd1 -eGFP mice immunoreactive for eGFP ( b ) and PlexinD1 ( c ). ( d – f ) Comparison of CR cells migration (arrows in d , e ) after incubation with SEAP ( d ) and Sema3E-AP ( e ) in E12.5 CH explants of Plxnd1 -eGFP. Quantifications of the experiments are shown in f . Plots show mean±s.e.m. SEAP ( n =14); Sema3-AP ( n =18). *** P <0.001, Student’s t -test. ( g , h ) Examples of identified CH-derived CR cells migration on SEAP ( g ) and Sema3E-AP ( h ) treated cultures. Each CR cell trajectory is labelled with a different colour line using the (ImageJ) software analysis. ( I , j ) Graph showing the trajectories of identified CR cells in the video time-lapse experiments. A total of 38 and 39 cells are plotted in i and j , respectively. ( k ) Histogram showing the total distance migrated in the video time-lapse experiments and the effect of the Sema3E-AP incubation. Data are represented by mean±s.e.m. of three different experiments. *** P <0.001 Student’s t -test. Scale bars, b =200 μm pertains to c . d =300 μm pertains to e , g and h . Full size image Sema3E or PlexinD1 absence increased CR cells migration Subsequently, we aimed to corroborate our previous observations in a closer in vivo paradigm, by transplanting the CH from Actin-eGFP in E13.5 Sema3E o/o mice or Sema3E +/+ telencephalic slices ( Fig. 3 ). After 24–36 h in culture, slices were processed to eGFP and CALR immunostaining. Results revealed a larger number of eGFP/CALR-positive cells migrated over the Sema3E o/o slices compared with Sema3E +/+ ( Fig. 3b–e ). More importantly, the number of migrating eGFP-positive CR cells ( Fig. 3f ) and the migrated distance ( Fig. 3g ) were considerably reduced in both Sema3E o/o and Sema3E +/+ slices treated with exogenous Sema3E-AP-containing media, when compared with their controls (% of decrease in number of migrating cells=46% ( Sema3E +/+ ) and 67% ( Sema3E o/o ); % of decrease in migrated distance=40% ( Sema3E +/+ ) and 38% ( Sema3E o/o )). Finally, we repeated the confrontation experiments by culturing CH from Sema3E +/+ (not shown) or Sema3E o/o with cortical meningeal cells ( Fig. 3h–l ). Results indicate that genetic ablation of Sema3E does not impair the chemoattraction on CR cells by meninges (PQ/DQ ratio=1.97±0.17, Fig. 3l ; mean±s.e.m.). However, the addition of Sema3E-AP to the media decreased the migrated distance (from 70.4±10 μm (+SEAP) to 36.4±4 μm (+Sema3E-AP), Fig. 3k ) and the chemoattraction (from 1.97±0.17 PQ/DQ (+SEAP) to 1.29±0.2 PQ/DQ (+Sema3E-AP), Fig. 3l )(Values are expressed as mean±s.e.m.). Finally, in order to determine whether PlexinD1 expressed by CR cells mediates these results, we analysed parallel CH cultures derived from Plxnd1 o/o or Plxnd1 +/+ mice confronted with cortical meningeal cells ( Fig. 4 ). Mice lacking Plxnd1 die around birth due to vascular defects [29] . Thus, prior to using these mice, we aimed to explore putative differences in the CH between Plxnd1 o/o and wild-type mice ( Supplementary Fig. 6 ). Non-radioactive in situ hybridization of E12.5 Plxnd1 o/o revealed the presence of Wnt2b -positive CH with anatomical characteristics similar to those of wild-type mice ( Supplementary Fig. 6a–c ). Next, CALR-immunoreacted sections during embryonic development demonstrated normal gross cytoarchitectonics in mutant embryos with the cortical plate, a marginal zone, and a well-defined subplate. In addition, immunopositive thalamocortical axons as well as CALR-positive tangentially migrating GABAergic interneurons were also observed in the intermediate-subventricular zone at E14.5 ( Supplementary Fig. 6d ). This normal development in the absence of PlexinD1 was also recently reported in Emx1 Cre -PlxnD1 Δ/flox embryos [31] . However, western blotting of CXCR4 expression demonstrated a decrease of ≈20% in the developing neocortex at E12.5 in Plxnd1 o/o mice compared with Plxnd1 +/+ or Plxnd1 +/o ( Supplementary Fig. 6e ). Next, we aimed to analyse the behaviour of CH-derived CR cells ( Plxnd1 o/o and Plxnd1 +/+ ) in collagen three-dimensional cultures. Video time-lapse recordings showed that Plxnd1 o/o CR cells showed enlarged leading neurites with low number of protrusions compared with Plxnd1 +/+ ( Supplementary movies 5,6 ); this behaviour correlates with a decrease in the migration speed compared with Plxnd1 +/+ (0.226±0.009 μm min −1 ; mean±s.e.m. ); Plxnd1 o/o (0.161±0.008 μm min −1 ; mean±s.e.m.). In parallel experiments, E12.5 CHs were confronted with cortical meningeal cells ( Fig. 4 ), CR cells lacking Plxnd1 were attracted by meningeal cells similarly to wild-type CR cells in three-dimensional hydrogels ( Fig. 4a,b,d ). However, the number of CR cells migrating out of the CH explants under the influence of meningeal cells was lower in knockout than in Plxnd1 +/+ or Plxnd1 +/o explants ( Fig. 4a–c ). Nevertheless, when Plxnd1 o/o cultures were treated with Sema3E-AP-conditioned media, there were no changes in the chemoattraction by meningeal cells ( Fig. 4b,d ) (PQ/DQ=1.7±0.2 (+SEAP) versus 1.5±0.29 (+Sema3E-AP) in Plxnd1 o/o explants). Values are expressed as mean±s.e.m.) ( Fig. 4 ). These data indicate that Sema3E/PlexinD1 signalling modulates the effects of the diffusible meningeal factor on CR cell behaviour by acting on its motogenic properties. 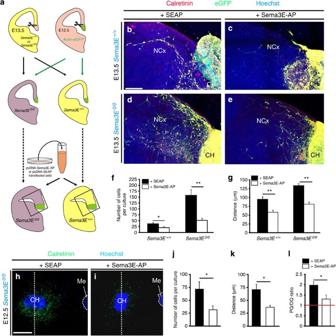Figure 3: Migration of CR cells is inhibited by Sema3E in brain slices. (a) Schematic representation of the assay. The boxed region inais shown in (b–e). eGFP-positive CH from Actin-eGFP embryos was transplanted in replacement of original hem ofSema3E+/+(b,c) andSema3Eo/o(d,e) E13.5 brain slices, which were further treated with SEAP (b,d) or Sema3E-AP (c,e) for 48 h in culture. Quantification of the number of CR cells identified as eGFP (green)/CALR (red)-positive cells exiting from the hem and migrated distance is shown in (f,g). The number of the eGFP-positive migrating cells (f) and the migrated distance (g) under each condition are plotted. Plots show mean±s.e.m.Sema3E+/+(number of cultures:+SEAP,n=9;+Sema3E-AP,n=7);Sema3Eo/o(number of cultures:+SEAP,n=10;+Sema3E-AP,n=8). (h,i) Distribution of hem-derived CR cells from E12.5Sema3Eo/oembryos confronted with meninges (Me) and treated with SEAP (h) or Sema3E-AP (i). Dotted lines indicate the border of the meningeal explant. (j–l) Quantification of the experiments in (h,i). The number of cell/culture and the distance is plotted. The proximal quadrant/distal quadrant (PQ/DQ) ratio is also shown in (l). Number of cultures:+SEAP, (n=15);+Sema3E-AP, (n=16). Plots show mean±s.e.m. *P<0.05, **P<0.01. Student’st-test. Scale bars, 200 μm inb–e; 300 μm inh,i. Figure 3: Migration of CR cells is inhibited by Sema3E in brain slices. ( a ) Schematic representation of the assay. The boxed region in a is shown in ( b – e ). eGFP-positive CH from Actin-eGFP embryos was transplanted in replacement of original hem of Sema3E +/+ ( b , c ) and Sema3E o/o ( d , e ) E13.5 brain slices, which were further treated with SEAP ( b , d ) or Sema3E-AP ( c , e ) for 48 h in culture. Quantification of the number of CR cells identified as eGFP (green)/CALR (red)-positive cells exiting from the hem and migrated distance is shown in ( f , g ). The number of the eGFP-positive migrating cells ( f ) and the migrated distance ( g ) under each condition are plotted. Plots show mean±s.e.m. Sema3E +/+ (number of cultures:+SEAP, n =9;+Sema3E-AP, n =7); Sema3E o/o (number of cultures:+SEAP, n =10;+Sema3E-AP, n =8). ( h , i ) Distribution of hem-derived CR cells from E12.5 Sema3E o/o embryos confronted with meninges (Me) and treated with SEAP ( h ) or Sema3E-AP ( i ). Dotted lines indicate the border of the meningeal explant. ( j – l ) Quantification of the experiments in ( h , i ). The number of cell/culture and the distance is plotted. The proximal quadrant/distal quadrant (PQ/DQ) ratio is also shown in ( l ). Number of cultures:+SEAP, ( n =15);+Sema3E-AP, ( n =16). Plots show mean±s.e.m. * P <0.05, ** P <0.01. Student’s t -test. Scale bars, 200 μm in b – e ; 300 μm in h , i . 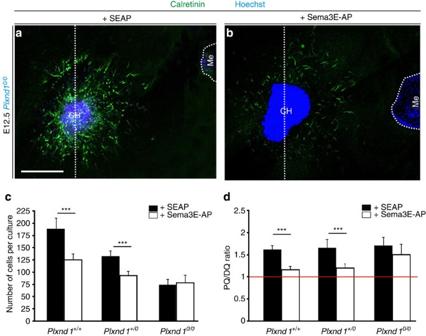Figure 4: PlexinD1 modulates the motogenic properties of hem-derived CR cells. (a,b) Migration of hem-derived CALR-positive CR cells (green) obtained fromPlxnd1o/oembryos confronted with meninges in the presence of SEAP (a) or Sema3E-AP (b). The quantification of experiments is shown in (c,d). Plots illustrate the number of cells per culture (c), and the PQ/DQ ratios (d) in the three different genotypes (Plxnd1+/+(number of cultures:+SEAP,n=18;+Sema3E-AP,n=27);Plxnd1+/o(number of cultures:+SEAP,n=28;+Sema3E-AP,n=33);Plxnd1o/o(number of cultures:+SEAP,n=19; Sema3E-AP,n=13)). Plots show mean±s.e.m. ***P<0.001, Student’st-test. Scale bars, 300 μm in (a,b). Full size image Figure 4: PlexinD1 modulates the motogenic properties of hem-derived CR cells. ( a , b ) Migration of hem-derived CALR-positive CR cells (green) obtained from Plxnd1 o/o embryos confronted with meninges in the presence of SEAP ( a ) or Sema3E-AP ( b ). The quantification of experiments is shown in ( c , d ). Plots illustrate the number of cells per culture ( c ), and the PQ/DQ ratios ( d ) in the three different genotypes ( Plxnd1 +/+ (number of cultures:+SEAP, n =18;+Sema3E-AP, n =27); Plxnd1 +/o (number of cultures:+SEAP, n =28;+Sema3E-AP, n =33); Plxnd1 o/o (number of cultures:+SEAP, n =19; Sema3E-AP, n =13)). Plots show mean±s.e.m. *** P <0.001, Student’s t -test. Scale bars, 300 μm in ( a , b ). Full size image Sema3E/PlexinD1 modulates CXCL12/CXCR4 signalling It is well established that CR cell migration is promoted by CXCL12/CXCR4 signalling [17] , [18] . Thus, we aimed to determine whether Sema3E/PlexinD1 might modulate the chemokine signalling ( Fig. 5 ). First, we co-cultured E12.5 CH explants (from C57BL/6J embryos) with CXCL12 expressing COS1 cell aggregates ( Fig. 5a–d ). Numerous CALR-positive CR cells migrated towards the CXCL12-secreting COS1 aggregate ( Fig. 5a,c ). In contrast, when explants were incubated with Sema3E-AP, this preferential migration was not observed ( Fig. 5b,c ). Thus, Sema3E-AP considerably reduced the number of migrating cells as well as the CXCL12-mediated CR cell migration. Next, we analysed whether the pharmacological ablation of CXCL12/CXCR4 signalling affected the Sema3E/PlexinD1-mediated effects on hem-derived CR cells confronted with cortical meningeal cells ( Fig. 5d ). We performed co-culture experiments of C57BL/6J CH and meninges in the presence or absence of both Sema3E and the CXCR4 inhibitor AMD3100 (10 μM) [18] , [32] , [33] . The combined treatment with AMD3100 and Sema3E-AP had similar effects to the addition of Sema3E-AP or AMD3100 alone ( Fig. 5d ). Indeed, in all cases, the chemoattractive effect exerted by meningeal cells was significantly reduced ( Fig. 5d ), suggesting that the two signalling mechanisms may run parallel. Vilz [34] indicated that Plxnd1 expression is selectively abrogated in pontine nuclei neurons in Cxcr4 o/o mice, in contrast to other cerebellar populations (for example, inferior olive) and forebrain neurons. So, in order to biochemically explore a putative interaction of the two signalling pathways, we used COS1-transfected cells ( Fig. 5 ; Supplementary Figs 7–10 ), because the levels of CXCR4 and PlexinD1 expression reached after transient transfection were sufficient to clearly characterize intracellular events. Indeed, the results indicated no differences in PlexinD1 ( Fig. 5e ) or Cxcr4 ( Fig. 5f ) expression under any experimental condition with western blotting and RT–qPCR, respectively. We observed that incubation with CXCL12 (50 μg ml −1 of culture media) on Cxcr4- transfected COS1 cells activated ERK1/2 kinases as described [35] ( Fig. 5g ; Supplementary Fig. 7 ). This activation, which peaked 5 minutes after CXCL12 incubation, was largely abolished after AMD3100 treatment, and was completely absent after U0126 incubation (10 μM) ( Fig. 5g , Supplementary Figs 7,8 ), irrespective of the expression of Plxnd1 . These data support the idea that PlexinD1 expression is not necessary for CXCL12/CXCR4 intracellular signalling in transfected cells (see also Fig. 4 ). Next, cells were co-transfected with Cxcr4 and Plxnd1 encoding plasmids and treated with CXCL12 in the presence or absence of Sema3E-AP ( Fig. 5h ; Supplementary Figs 9–12 ). In these experiments, we observed a clear delay in ERK1/2 activation (which peaked at 30 min) in the presence of Sema3E-AP ( Fig. 5h , Supplementary Fig. 9 ). In addition, previous reports have indicated that PlexinD1 signalling acts on the F-Actin cytoskeleton due to its GAP activity (see ref. 36 for review). Therefore, we aimed to explore whether Sema3E modified the activity of ADF/Cofilin, a well-described F-Actin-depolymerizing factor under the control of LIM kinases ( Fig. 5h , Supplementary Fig. 10 ). Revealed blots showed a considerable increase in phospho-Cofilin in CXCL12 stimulated double ( Cxcr4/Plxnd1 ) co-transfected cells after Sema3E-AP treatment ( Fig. 5h , Supplementary Fig. 10 ). Moreover, to determine whether the intracellular GAP domain is the responsible of the observed results, we repeated the experiments in double transfected cells with Cxcr4/Plxnd1-ΔGAP ( Fig. 5h , Supplementary Figs 11,12 ). Immunoreacted blots indicated that Cxcr4/Plxnd1 -Δ GAP -transfected cells showed a timecourse activation of pERK1/2 and ADF/Cofilin phosphorylation after Sema3E-AP treatment similar to SEAP treatment ( Fig. 5h , Supplementary Figs 11,12 ). In addition, these results were similar to previously observed after SEAP treatment in ( Cxcr4/Plxnd1 ) co-transfected cells ( Fig. 5h ; Supplementary Fig. 12 ). Thus, the delay observed in pERK1/2 and ADF/Cofilin induced by Sema3E depends of the presence of the integrity and associated functions of cytoplasmic tail of PlexinD1. It has been reported that, increased phosphorylation of ADF/Cofilin leads to a decreased number of free barbed ends to initiate actin polymerization for actin-based protrusion processes required for correct chemotaxis [37] . Indeed, in vitro video time-lapse imaging experiments demonstrates that CR cells incubated with Sema3E-AP showed a fast decrease in branches of the leading neurites compared with SEAP-treated cells, which correlates with lower cell migration and soma movement ( Supplementary Fig. 13 , Supplementary movie 7 ). Taken together, our results indicate that Sema3E/PlexinD1 signalling might modulate the activation of both ERK1/2 pathways and ADF/Cofilin in the presence of CXCL12, reducing the motogenic properties of CR cells. 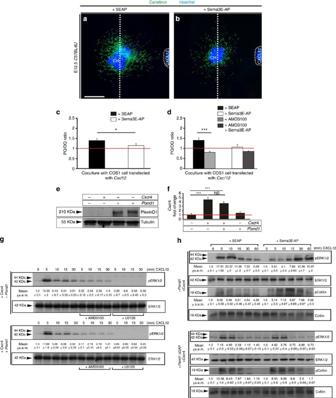Figure 5: Sema3E modulates CXCL12-mediated chemoattraction. (a,b) Migration of CR cells confronted with COS1 cell aggregates expressing CXCL12 in presence of SEAP (a) or Sema3E-AP (b). The PQ/DQ ratio is shown inc. (number of cultures:+SEAP,n=24;+Sema3E-AP,n=48). (d) Quantification of the dispersion of hem-derived CR cells confronted with meninges in the presence of SEAP or Sema3E-AP and the CXCR4 inhibitor AMD3100 (number of cultures: SEAP,n=12, SEAP+AMD3100,n=16; Sema3E-AP,n=12; Sema3E+AMD3100,n=11). (e,f) Expression level of PlexinD1 determined by western blotting (e) andCxcr4transcript levels determined by RT–qPCR (f) in COS1 cells transfected withPlxnd1and/orCxcr4.Tubulin is included as loading control ine. (g) Time course of ERK1/2 activation by CXCL12 in COS1 cells transfected withPlxnd1encoding plasmids in the presence of AMD3100 or U0126. PlexinD1 was not necessary for the intracellular signalling mediated by CXCL12/CXCR4 in COS1 cells. (h) Effects of Sema3E-AP treatment on CXCL12-mediated signalling in COS1 cells co-transfected withCxcr4andPlxnd1orPlxnd1-ΔGAP. Each experiments assay was performed three times and the quantification of each band was shown below each blot as mean±s.e.m. Plots show mean±s.e.m. Student’st-test, *P<0.05, ***P<0.001. Scale bars, 300 μm inapertains tob. Figure 5: Sema3E modulates CXCL12-mediated chemoattraction. ( a , b ) Migration of CR cells confronted with COS1 cell aggregates expressing CXCL12 in presence of SEAP ( a ) or Sema3E-AP ( b ). The PQ/DQ ratio is shown in c . (number of cultures:+SEAP, n =24;+Sema3E-AP, n =48). ( d ) Quantification of the dispersion of hem-derived CR cells confronted with meninges in the presence of SEAP or Sema3E-AP and the CXCR4 inhibitor AMD3100 (number of cultures: SEAP, n =12, SEAP+AMD3100, n =16; Sema3E-AP, n =12; Sema3E+AMD3100, n =11). ( e , f ) Expression level of PlexinD1 determined by western blotting ( e ) and Cxcr4 transcript levels determined by RT–qPCR ( f ) in COS1 cells transfected with Plxnd1 and/or Cxcr4. Tubulin is included as loading control in e . ( g ) Time course of ERK1/2 activation by CXCL12 in COS1 cells transfected with Plxnd1 encoding plasmids in the presence of AMD3100 or U0126. PlexinD1 was not necessary for the intracellular signalling mediated by CXCL12/CXCR4 in COS1 cells. ( h ) Effects of Sema3E-AP treatment on CXCL12-mediated signalling in COS1 cells co-transfected with Cxcr4 and Plxnd1 or Plxnd1-ΔGAP . Each experiments assay was performed three times and the quantification of each band was shown below each blot as mean±s.e.m. Plots show mean±s.e.m. Student’s t -test, * P <0.05, *** P <0.001. Scale bars, 300 μm in a pertains to b . Full size image CR cell migration in Sema3E o/o and Plxnd1 o/o -mutant mice The above results suggest deficits in CR cell migration in mice lacking Sema3E/PlexinD1 signalling as demonstrated in the Cxcr4 o/o mice (see refs 18 , 38 ). However, although exhibiting defects in emotional behaviour and working memory, Sema3E o/o mice develop to adulthood [30] , in contrast to Plxnd1 o/o mice. Thus, we analysed in detail the distribution of CR cells in Sema3E o/o and Plxnd1 o/o in the marginal zone/layer I of the medial cortex and hippocampus at perinatal stages ( Fig. 6 ). Deficits in Cxcr4 lead to changes in granule cell layer formation in developing hippocampus [39] . First, we explored differences in the number of granule cells (Prox-1 positive) as well as CR cells (CALR positive) in the hippocampus of Sema3E o/o mice. Neither experiments revealed differences in the total number of granules or CR cells between Sema3E o/o and Sema3E +/+ mice ( Fig. 6a–d,g,h ). Next, in situ hybridization experiments determined that Reln -positive CR cells were localized in the slm/ml of both Plxnd1 o/o and wild-type hippocampus at E18.5 without the presence of ectopically located cells in the stratum radiatum as observed in Cxcr4 o/o mice [18] , [38] ( Fig. 6e,f ). In fact, cell counts showed no statistically significant differences in Reln -positive cells between Plxnd1 o/o and Plxnd1 +/+ in the hippocampus and the medial cortex ( Fig. 6i ). However, cell counts performed throughout marginal zone of Plxnd1 o/o and Plxnd1 +/+ mice revealed higher numbers of Reln -positive CR cells in the medial cortical regions (retrosplenial cortex) in Plxnd1 +/+ than in Plxnd1 o/o mice ( Fig. 6j–l ). These data suggest that, in the absence of Sema3E/PlexinD1 signalling, hem-derived CR cells reached more dorsal neocortical regions ( Fig. 7 ). 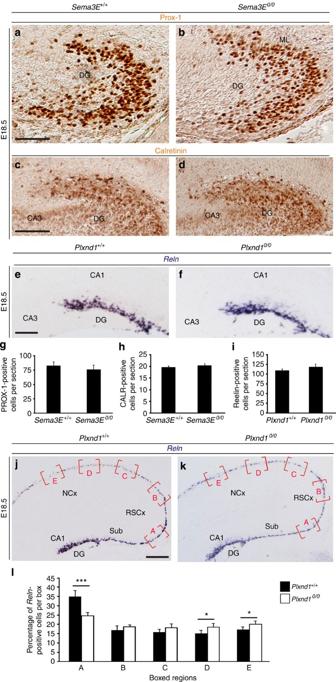Figure 6: Analysis ofSema3Eo/oandPlxnd1o/ohippocampus and medial cortex. (a–f) Photomicrographs illustrating the distribution of Prox-1 immunoreactive granule cells (a,b) and CALR-positive elements (c,d) in the slm/ml inSema3E+/+(a,c) andSema3Eo/o(b,d) E18.5 hippocampus. Quantification of the experiments is shown ingandh(Sema3E+/+embryosn=8 andSema3Eo/on=10). No differences were observed between genotypes in Prox-1 and CALR immunostaining. (e,f) Low power photomicrographs illustrating the distribution ofRelnin the hippocampus ofPlxnd1+/+(e) andPlxnd1o/o(f) E18.5 embryos from the same litter. Quantification of the number ofReln-positive CR cells in the slm/ml is shown ini(Plxnd1+/+embryosn=7 andPlxnd1o/on=6). No statistical differences in the numbers of CR cells were seen between genotypes. (j–l) Low power photomicrograph (j,k) and quantification (l) (Plxnd1+/+embryosn=7 andPlxnd1o/on=6) of the number of Reelin-positive CR cells in five different boxes (200 μm width) throughout marginal zone inPlxnd1+/+(j) andPlxnd1o/o(k). Notice that inPlxnd1+/+34.9% of CR cells were located in the retrosplenial cortex (boxa) in contrast to 24.8% inPlxnd1o/o. Plots show mean±s.e.m. Student’st-test, *P<0.05, ***P<0.001. Scale bars, 200 μm ina–d; 200 μm ine,f,j,k). Figure 6: Analysis of Sema3E o/o and Plxnd1 o/o hippocampus and medial cortex. ( a – f ) Photomicrographs illustrating the distribution of Prox-1 immunoreactive granule cells ( a , b ) and CALR-positive elements ( c , d ) in the slm/ml in Sema3E +/+ ( a , c ) and Sema3E o/o ( b , d ) E18.5 hippocampus. Quantification of the experiments is shown in g and h ( Sema3E +/+ embryos n =8 and Sema3E o/o n =10). No differences were observed between genotypes in Prox-1 and CALR immunostaining. ( e , f ) Low power photomicrographs illustrating the distribution of Reln in the hippocampus of Plxnd1 +/+ ( e ) and Plxnd1 o/o ( f ) E18.5 embryos from the same litter. Quantification of the number of Reln -positive CR cells in the slm/ml is shown in i ( Plxnd1 +/+ embryos n =7 and Plxnd1 o/o n =6). No statistical differences in the numbers of CR cells were seen between genotypes. ( j – l ) Low power photomicrograph ( j , k ) and quantification ( l ) ( Plxnd1 +/+ embryos n =7 and Plxnd1 o/o n =6) of the number of Reelin-positive CR cells in five different boxes (200 μm width) throughout marginal zone in Plxnd1 +/+ ( j ) and Plxnd1 o/o ( k ). Notice that in Plxnd1 +/+ 34.9% of CR cells were located in the retrosplenial cortex (box a ) in contrast to 24.8% in Plxnd1 o/o . Plots show mean±s.e.m. Student’s t -test, * P <0.05, *** P <0.001. Scale bars, 200 μm in a – d ; 200 μm in e , f , j , k ). 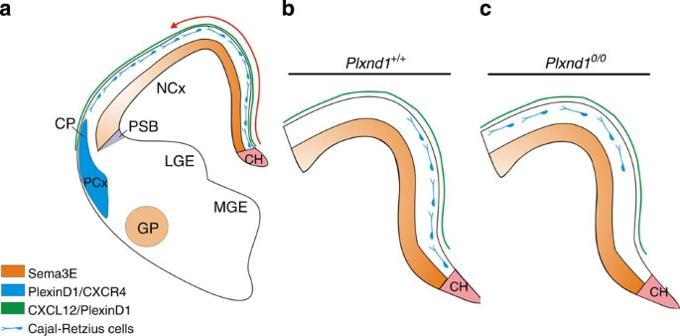Figure 7: Proposed role of Sema3E/PlexinD1 in CR cells migration. (a) Cross-sectional diagrams illustrating the pattern of expression of Sema3E, PlexinD1, CXCL12 and CXCR4 in neural elements at E12.5. (b,c) Diagrams illustrating the location of CR cells in dorsomedial cortex (b,c) with functional Sema3E/PlexinD1 signalling (b) and in absence of Sema3E/PlexinD1 signalling (c). In the diagrams only two different cohorts of postmitotic CR cells are indicated in violet and blue. As indicated in the manuscript, with functional Sema3E/PlexinD1 signalling (b) the migratory properties of CR cells remained unaltered and they migrated following the described tangential routes (red arrow ina) towards dorsal cortex (b). In contrast, in the absence of Sema3E/PlexinD1 (c), although a whole population of CR cells migrated along preplate, they reached more dorsomedial regions. CP, cortical plate; GP, globus pallidus; LGE, lateral ganglionic eminences; MGE, medial ganglionic eminences; NCx, dorsal neocortex; PSB, pallial–subpallial boundary.Fig. 1. Full size image Figure 7: Proposed role of Sema3E/PlexinD1 in CR cells migration. ( a ) Cross-sectional diagrams illustrating the pattern of expression of Sema3E, PlexinD1, CXCL12 and CXCR4 in neural elements at E12.5. ( b , c ) Diagrams illustrating the location of CR cells in dorsomedial cortex ( b , c ) with functional Sema3E/PlexinD1 signalling ( b ) and in absence of Sema3E/PlexinD1 signalling ( c ). In the diagrams only two different cohorts of postmitotic CR cells are indicated in violet and blue. As indicated in the manuscript, with functional Sema3E/PlexinD1 signalling ( b ) the migratory properties of CR cells remained unaltered and they migrated following the described tangential routes (red arrow in a ) towards dorsal cortex ( b ). In contrast, in the absence of Sema3E/PlexinD1 ( c ), although a whole population of CR cells migrated along preplate, they reached more dorsomedial regions. CP, cortical plate; GP, globus pallidus; LGE, lateral ganglionic eminences; MGE, medial ganglionic eminences; NCx, dorsal neocortex; PSB, pallial–subpallial boundary. Fig. 1 . Full size image In this study, we have shown that Sema3E has the capacity to modulate the migration of PlexinD1-positive CR cells triggered by CXCL12/CXCR4 signalling [17] , [18] . Chemokine signalling through CXCL12/CXCR4 is a common mechanism controlling the migration of several cell types along the body axis, such as hematopoietic progenitor cells [40] , vascular endothelial cells [41] , melanocytes [42] and tumour cells [43] , [44] . In addition to the present results, it has been reported that in the CNS, in addition to CR cells, the migration of cerebellar granule precursors [34] , cortical interneurons [23] , microglia [45] , neural precursor cells [46] , and certain brain tumour cells [33] is also dependent on CXCL12/CXCR4 signalling. In addition, Semaphorins and their classic receptors (Plexins and Neuropilins) have been associated primarily with multiple functions, including cell migration and axon chemotaxis (for review see ref. 47 ). In particular, Sema3E and PlexinD1 have been reported to play an active role in vascular system development [29] , [48] , [49] , but they also control the migration of mouse thymocytes [50] and tumour cells [51] . Indeed, mice lacking Plxnd1 showed impaired thymocyte trafficking [50] and a poorly developed vascular system [29] . Today, it is generally accepted that the stereotypical organization of the blood vessels is guided by the same genetic and molecular mechanisms that guide developing axons (reviewed in refs 26 , 36 ), although it is only in recent years that the developmental role played by Sema3E/PlexinD1 in the central and peripheral nervous systems began to be elucidated. For example, Sema3E/PlexinD1 signalling controls the development of several axonal projections in the developing mouse telencephalon [30] as well as the establishment of glutamatergic synapse formation [52] , and it triggers axonal growth cone inhibition [53] . In fact, some of these effects are mediated by the interaction of the VEGF receptor type 2 (VEGFR2 or Flk-1) with PlexinD1 and Neuropilin1 (ref. 28) [28] . However, to our knowledge, this is the first report describing the role of Sema3E/PlexinD1 in controlling murine CR cell migration via modulation of CXCL12/CXCR4 signalling. The present data also correlate with a study by Holl et al. [54] , who demonstrated that Plxnd1 o/o B cells showed decreased migration induced by CXCL12 and other chemokines. However, as regards their migratory behaviour, CR cells lacking Sema3E/PLexinD1 signalling migrated correctly through the preplate and remained confined in the hippocampal slm/ml and in the marginal zone/layer I of the neocortex. This fact, together with our in vitro experiments, strongly indicates that Sema3E/PlexinD1 does not play a chemotactic role in CR cells. In fact, neither PlexinD1 nor Sema3E is necessary for correct CXCL12/CXCR4 signalling (at least in transfected COS cells). PlexinD1 acts as a RasGAP to antagonize PIK3 signalling and integrin-mediated cell adhesion to the extracellular matrix [53] , [55] . In fact, a small GTPase Rnd2 was found to bind PlexinD1 in embryonic ventrolateral cortex neurons, to reduce Ras activity and induce growth cone collapse [53] . In addition, it has been recently described that motogenic effects of CXCL12 in neural progenitors are mediated by PI3K [46] which may support a role for PlexinD1 (antagonizing PIK3 signalling) in modulating the motogenic properties of CR cells under the influence of CXCL12. Thus, with the present data, we cannot rule out the possibility that the inhibitory effect of Sema3E/PlexinD1 may act in parallel to CXCL12/CXCR4 activity by modulating the interaction of integrins at the CR cells and the extracellular matrix, which in turn may delay the activation of ERK1/2; considering that, it has been described that CXCL12/CXCR4 mediates its action by integrins in other cell types [56] . In fact, these inhibitory effects on cell spreading have also been described for other Plexins (for example, Sema4D/PlexinB1 (ref. 57) [57] ). Thus, when activated, PlexinB1 also elicits the disassembly of focal contacts and inhibits cell spreading. In our experiments, Sema3E delayed ERK1/2 activity mediated by CXCL12/CXCR4 and increased the phosphorylation of ADF/Cofilin, which affect the dynamics of the leading edge of CR cells and their migration. These effects are mediated by the GAP domain of PlexinD1. Furthermore, Sema3E/PlexinD1 binding mediates the disassembly of actin filaments by PAK activation by modulating the activity of small GTPases in several cell types (see ref. 36 for review). In this sense, it has been widely demonstrated that RHO/PAK/LIMK/Cofilin signalling is critical in growth cone collapse by secreted Semaphorins. Also, the positive involvement of CXCL12 in migration by LIMK activation in Jurkat cells has been previously described [58] . In conclusion, our data suggest that both Sema3E and CXCL12 might cooperate in controlling the activity of ADF1/Cofilin and the intracellular signalling effects of CXCL12/CXCR4 on COS1 cells and most probably on CR cells. Thus, although other factors could be involved, the absence of Sema3E/PlexinD1 signalling in CR cells induces an unbalanced control of the actin cytoskeleton and probably binding to the extracellular matrix, leading to increased migration and cell spreading in marginal zone/layer I in vivo ( Fig. 7 ). Our data also corroborate recent results of Deck et al. [31] , in axon guidance showing that in the absence of Sema3E , corticothalamic axons enter prematurely into the subpallium. In fact, guidance of migrating neurons shares many features with axonal guidance, as well as with vascular development from the use of substrates to the specific cues regulating chemotaxis [22] . On the other hand, the expression of a second receptor of CXCL12 (CXCR7) has been reported in CR cells [59] . Thus, we cannot rule out that Sema3E/PlexinD1 may also act on CXCR7 functions on CXCR4-mediated chemoattraction in CR cells as indicated [59] similarly as happens in subventricular cells in the rostral migratory stream [59] or cortical interneurons [60] . In fact, current experiments of our laboratory are exploring this challenging hypothesis. In a broad sense, the effects of Sema3E/PlexinD1 on axon guidance can be categorized as inhibitory (present results, see also refs 30 , 53 , 55 , 61 ) or attractive [30] , [61] , depending on the presence of co-receptors Neuropilin 1 and VEGFR2, but more importantly on specific binding partners in the PlexinD1 cytoplasmic tail (see refs 28 , 36 , 62 for reviews). Neither Neuropilin 1 nor 2 is expressed by CR cells [63] ; this is restricted to the principal cortical neurons [64] , [65] . In addition, VEGFR2 or VEGF are also expressed by developing neurons in the neocortex as well as within the vascular structures of meninges, but not by CR cells [66] . Thus, under these expression patterns, the negative effects of Sema3E/PlexinD1 signalling may occur in CR cells lacking both Neuropilin1 and VEGFR2 (see also ref. 30 for details). A recent study reported that the distribution of CR cells is also mediated by radial glial cells [67] . Indeed, an absence of radial glia results in local displacement of CR cells in layer I [67] . In addition, the expression of Sema3E by radial glia at the subpallium in the lateral ganglionic eminence has been recently suggested [31] . In our study, we observed relevant but also specific expression of Sema3E mRNA in E12.5-E13.5 mice neocortex. Late in development, Sema3E is expressed by cortical plate neurons in the most caudolateral cortical regions. In fact, Sema3E can be detected in the upper half portion of the neocortex by western blot techniques ( Supplementary Fig. 3 ). However, with present data, we cannot clearly determine the neocortical cells responsible for Sema3E expression at these embryonic stages, since the cell definition level of the in situ hybridization signal is poor, and the commercially available antibodies only label Sema3E in western blot techniques or in human-derived tissues. Nevertheless, the close relationship between CR cells and the radial glia scaffold has previously been described (see for review; ref. 1 ) and a molecular interaction between radial glia on CR cells controlling their tangential migration seems reasonable given the present data. In conclusion, in the absence of Sema3E/PlexinD1 signalling, the correct migration of CR cells is not fully modulated in the preplate/marginal zone ( Fig. 7 ). Whether Sema3E/PlexinD1 signalling is enhanced in parallel with the recently described contact-mediated migration of CR cells is a question that warrants further study. In this sense, we cannot also rule out the possibility that haemophilic interactions between PlexinD1 expressed by CR [14] may play a role in contact-mediated migration of CR cells, as happens with members of the plexin B subfamily (Plexin B3) [68] . The functions of CR cells modulating migration of cortical plate neurons seemed to remain unaltered in the absence of Sema3E/PlexinD1 signalling (see Fig. 6 ). However, whether these differences in migration may modify other CR cell functions (for example, modulating specific axon elongation) is unknown, and also warrants further study. Nevertheless, our data describing for the first time a role for Sema3E/PlexinD1 in CR cells reinforce the notion that the vascular and nervous systems share molecular mechanisms controlling cell migration during development. Animals Plxnd1 +/o and Sema3E +/o mice were reported in ref. 29 . Mice were maintained in heterozygous genotype and experiments were performed using embryos of the three different genotypes. Animals were genotyped by PCR, as previously described elsewhere [29] . Plxnd1-eGFP mice were obtained from the Mutant Mouse Regional Resource Center (MMRRC; University of California, CA, USA). Actin-eGFP and C57BL/6J mice were purchased from Jackson Laboratories (Bar Harbor, ME, USA). Animals were maintained in a pathogen-free barrier facility at the University of Barcelona animal facility. Experiments were approved by the University of Barcelona Animal Care and Use Committee and used in accordance with Spanish (RD223/88) and European (86/609/ECC) regulations. Analysis of enriched genes in the slm/ml of perinatal mice Newborn C57BL/6J pups were anaesthetized by hypothermia, their brains were aseptically removed and the hippocampus and the entorhinal cortex were dissected out. Using a McIIwain II tissue chopper, tissue pieces were cut into single horizontal sections (200–250 μm thick) containing both the entorhinal cortex and the hippocampus, and maintained in Hanks Balanced Salt Solution (Invitrogen, Carlsbad, CA, USA) containing 6.5 mg ml −1 glucose. The CA1 was dissected out and the slm of the CA1 was further isolated with a tungsten knife under microscope observation. A total of 400 pieces of the slm/ml from 50 pups from six different litters were obtained. Total RNA from the slm/ml and the rest of the CA1 were extracted with the miRVana isolation kit (Ambion, Austin, TX, USA) and quantified with a NanoDrop ND-1000 spectrophotometer, followed by quality assessment with the 2100 Bioanalyzer (Agilent Technologies), according to the manufacturer’s instructions. Acceptable quality values were in the 1.8–2.2 range for A260/A280 ratios, >0.9 for the rRNA ratio (28S/18S) and >8.0 for RIN (RNA Integrity Number). For RT–qPCR, purified RNAs were used to generate the corresponding cDNAs, which served as PCR templates for the mRNA quantification. The primers used in this study for RT–qPCR validation were the following: Reln: forward: 5′-CCATACTGCGGCCATGACTG-3′; reverse: 5′-CACCTGGTTGTCCATGTGAG-3′; Plxnd1: forward: 5′-CAGTTTGACCCCATGGATCCT-3′, reverse: 5′-TGGAGTGTACCTCACACGCC-3′; Gdf5 : forward: 5′-TGCCCCTGACTTAGGACAGAG-3′, reverse: 5′-ACACCATAGATATGACCCCCTG-3′. PCR amplification and detection were performed with the Roche LightCycler 480 detector, using 2 × SYBR Green Master Mix (Roche Farma Barcelona, Spain) as a reagent, following the manufacturer’s instructions. The reaction profile was as follows: denaturation–activation cycle (95 °C for 10 min) followed by 40 cycles of denaturation–annealing–extension (95 °C, 10 min; 72 °C, 1 min; 98 °C, continuous). mRNA levels were calculated using the LightCycler 480 software. The data were analysed using the ΔΔ C t method, which provides the target gene expression values as fold changes in the problem sample compared with a calibrator sample. Both problem and calibrator samples were normalized with the relative expression of a housekeeping gene (glyceraldehyde-3-phosphate dehydrogenase). Explant cultures The embryonic CH explants from E12.5 embryos were dissected out and placed in three-dimensional hydrogels (Matrigel, BD Bioscience, San Jose, CA, USA). They were cultured at 37 °C, 5% CO 2 and 95% humidity in Neurobasal medium supplemented with B27 (Invitrogen) and glucose (6.5 mg ml −1 ). After 2 days in vitro , genotypically identified cultures were paraformaldehyde fixed and processed. The number of cells that migrated out of the explants was counted, and the maximum distance migrated was also determined using a millimetric eyepiece in an Olympus IX71 inverted microscope. For cell confrontation assays, transfected COS1 cell (ATCC, code: CRL-1650. LGC Standards, Barcelona, Spain) aggregates expressing SEAP, Sema3A-myc , Sema3F, Sema3E-AP, Sema3E-myc or Cxcl12 were confronted with CH explants in Matrigel matrices. The Cxcl12 cDNA was obtained from ImaGenes (no. 3483088; accession number: BC006640). The Sema3E-AP, Sema3E-myc plasmids were provided by F. Mann. Sema3A-myc, Sema3F-myc , and SEAP- expressing vectors were a gift from Profs A. Chedotal and E. Soriano. Slice cultures Brain slices were obtained from E13.5 Sema3E o/o and Sema3E +/+ mice and CH from E12.5 Actin-eGFP mouse embryos. Slices were transferred to collagen-coated culture membrane (Millipore, Billerica, MA, USA) in 1.2 ml of medium (BME-F12 1:1, glutamine, 5% horse serum, penicillin and streptomycin (Invitrogen), 5% bovine calf serum (SAFC Biosciences, Lanexa, VA, USA)). The CH from wild-type or Sema3E o/o slices was discarded and replaced by the hem from Actin-eGFP mice embryos. After several hours, the medium was changed to Neurobasal medium supplemented as above and cultured for up to 48 h before analysis. Time-lapse analysis of CR cell migration We prepared CH explants as above in Fluorodish cell culture dishes (World Precision Instruments, Sarasota, FL, USA) and 8 h later, we performed the time-lapse analysis. To study cell migration, we transferred the culture dishes to an LCI system (Live Cell Instruments, Seoul, South Korea) for 24 h. After time-lapse recording, identified CR cells were selected in the last frames and their location in the x / y axis during these 24 h was plotted in the software. Indeed, the trajectory of these cells migrating into the hydrogel was also determined. The multi-tracking analysis was performed with the ImageJ software using the plugin mTrackJ (Biomedical Imaging Group Rotterdam of the Erasmus MC-University Medical Center Rotterdam, Netherlands). Tracking was performed in an inverted Olympus microscope IX71 ( × 20 objective) and images (5 megapixels resolution) were captured by an Olympus XC-50 camera (288 frames, 1 frame every 5 min). Cell tracking allows the analysis of the scrolling speed and position frame, (Xt, Yt). The cell position for each frame (position pixel) was determined with the Chemotaxis and migration Tool developed by G. Trapp and E. Horn (Ibidi, Germany) as plugin for ImageJ software. Antibodies and fluorochromes The following antibodies were used: rabbit anti-CALR (1:4,000; Swant, Marly, Switzerland), anti-PlexinD1 antibody (1:500; R&D Systems, Minneapolis, MN, USA), and anti-Reelin (1:300, Abcam, Cambridge, UK) and anti-GFP (1:1,000; Molecular Probes, Leiden, Netherlands). Rabbit anti-Prox-1 (1:2,000; Millipore) was used to identify granule cells in the hippocampus. Hoechst (1:200) was purchased from Sigma-Aldrich (St Louis, MO, USA). Propidium iodide (2.5 μg ml −1 , Sigma-Aldrich) was used to test the viability of explants. Alexa Fluor 488 goat anti-mouse and Alexa Fluor 568 goat anti-rabbit secondary antibodies were purchased from Molecular Probes. For western blots, we used an anti-PlexinD1 antibody (1:500) from R&D Systems; Cofilin (1:1,000), Cofilin phospho-Serine 3 (1:500); ERK phospho-threonine 202 /phospho-tyrosine 204 (pERK1-2) (1:500) antibodies were from Cell Signaling Technology (Beverly, MA, USA). Total ERK antibody (1:500) was from Transduction Laboratories (Lexington, KY, USA). Tubulin (1:10,000) was from Sigma and CXCR4 (1:500) from Acris Antibodies (Herford, Germany). Actin (1:5,000) was from Millipore. Goat anti-mouse horseradish peroxidase (HRP), goat anti-rabbit-HRP and rabbit anti-goat-HRP secondary antibodies were from DAKO (Glostrup, Denmark). Immunohistochemistry and in situ hybridization In situ hybridization was carried out as described previously [69] on 20 μm frozen brain sections of E12.5, E18.5 embryos, and in whole mount preparations. Both sense and antisense riboprobes were labelled with digoxigenin according to the manufacturer's instructions (Roche Farma). The following cDNA probes were used in this study: Reln (a gift from Tom Curran), Sema3E and PlexinD1 (a generous gift from Dr A. Kolodkin) and Wnt2b (kindly provided by P. Bovolenta). For immunohistochemistry studies of frozen brain sections, tissue was incubated with primary antibodies overnight, followed by appropriate secondary antibodies. Fluorescent staining was counterstained with Hoechst (Sigma-Aldrich). For immunohistochemistry studies of CH explants, cultures were fixed for 1 h in 4% buffered paraformaldehyde, incubated in 2% bovine serum albumin and 1% Triton X-100 in phosphate-buffered saline (PBS) for 4–6 h at room temperature, and subsequently incubated with primary antibodies for 48 h at 4 °C. After washing, appropriate fluorescent secondary antibodies were used and immunoreacted explants were mounted in Mowiol. Binding assay Sema3A-AP and control AP binding were performed essentially as described [30] . Mouse brains from E12.5 were frozen on dry ice, sectioned on a cryostat at 20 μm and fixed in methanol at −80 °C for 5 min. The sections were stored at −80 °C until use. After rehydrating the sections in PBS, they were overlaid with 1 nM Sema3E-AP diluted in Hanks Balanced Salt Solution (HBSS) and 20% fetal calf serum for 90 min, washed and fixed in 3.7% paraformaldehyde. Endogenous phosphatase was heat-inactivated at 65 °C. The AP fusion proteins were viewed through an enzymatic reaction with a solution containing 34 mM ml −1 of nitroblue tetrazolium and 18 mM ml −1 of 5-bromo-4chloro-3-indolylphosphate. Cell cultures To obtain a concentrated medium, COS1 cells were transfected with Sema3E-AP, Sema3A-myc, Sema3F or SEAP expression vectors. Forty-eight hours after transfection, the medium was collected and concentrated 1:10 in Millipore columns (with Ultracel-30 membrane), and protein was used 1:20 v/v in cultures. Results obtained using Sema3E-AP-containing media were corroborated in control experiments using 400–500 ng ml −1 of recombinant mouse Sema3E-Fc protein (cat. 3238-S3-025, R&D Systems). For time course analyses, COS1 cells were transfected with Cxcr4 ImaGenes (3592479; accession number: BC031665) and Plxnd1 or Plxnd1-ΔGAP . PlexinD1 and CXCR4 expression was determined by western blotting and Cxcr4 expression using RT–qPCR. RT–qPCR was performed on total RNA extracted from transfected COS1 with the miRVana isolation kit (Ambion). Purified RNAs were used to generate the corresponding cDNAs, which served as PCR templates for the mRNA quantification. The primers used in this study for RT–qPCR validation were the following Cxcr4 : forward: 5′-AACGTCCATTTCAATAGGATCT-3′, reverse: 5′-TTAGCTGGAATGAAAACTCGA-3′; Tubulin : forward: 5′-TTGGCCAGATCTTTAGACCAGACAAC-3′, reverse: 5′-CCGTACCACATCCAGGACAGAATC-3′. PCR amplification and detection were performed with the Roche LightCycler 480 detector, using 2 × SYBR Green Master Mix (Roche) as a reagent, following the manufacturer’s instructions. The reaction profile was as follows: denaturation–activation cycle (95 °C for 10 min) followed by 40 cycles of denaturation–annealing–extension (95 °C, 10 min; 72°C, 1 min; 98 °C, continuous). mRNA levels were calculated using the LightCycler 480 software. The data were analysed using the ΔΔ C t method. Samples were normalized by the relative expression of the housekeeping gene Tubulin . Twenty-four hours after transfection, COS1 cells were serum starved overnight, and then stimulated at different time points with CXCL12 (50 μg ml −1 ; Peprotech, Rocky Hill, NJ, USA) in the presence or absence of Sema3E-AP or SEAP concentrated media (as above). For CXCR4 receptor-blocking experiments, AMD3100 (Sigma-Aldrich) or MEK inhibitor U0126 (Promega, Fitchburg, WI) were added to the medium at a final concentration of 10 μM; control cultures received identical volumes of vehicle solution (0.1 M PBS) 30 min before stimulation with CXCL12. Statistics Data in this manuscript are expressed as mean±s.e.m. of at least three independent experiments. Means were compared using the two-tailed unpaired Student’s t -test. * P <0.05, ** P <0.01 and *** P <0.001, respectively. A P- value of <0.05 was considered statistically significant. How to cite this article : Bribián, A. et al. Sema3E/PlexinD1 regulates the migration of hem-derived Cajal-Retzius cells in developing cerebral cortex. Nat. Commun. 5:4265 doi: 10.1038/ncomms5265 (2014).